Orbital switching in a frustrated magnet The orbital is one of the four fundamental degrees of freedom in a solid, besides spin, charge and lattice. In transition metal compounds, it is usually the d orbitals which play deciding roles in determining the crystallographic and physical properties. Here we report the discovery of a unique structural transition in single crystals of the spin-1/2 quasi-kagomé antiferromagnet volborthite, Cu 3 V 2 O 7 (OH) 2 ·2H 2 O, whereby the unpaired electron 'switches' from one d orbital to another upon cooling. This is not a conventional orbital order–disorder transition, but rather an orbital switching that has not previously been observed. The structural transition is found to profoundly affect the magnetic properties of volborthite, because magnetic interactions between Cu spins in the kagomé lattice are considerably modified by the orbital switching. This finding provides us with an interesting example to illustrate the intimate interplay between the orbital degree of freedom and competing magnetic interactions in a frustrated magnet. Geometrical frustration in antiferromagnets has proven an attractive subject in condensed matter physics during the last few decades. When spins reside on the vertices of lattices consisting of triangles and interact antiferromagnetically, conventional magnetic long-range order (that is, Neel order) tends to be suppressed owing to the inability of the system to satisfy all interactions simultaneously—in other words, geometrical frustration. It is theoretically predicted that a fluctuating quantum-mechanical liquid state is realized at T =0 for many such systems [1] . These spin liquid states have, however, not yet been clearly observed in experiments, mainly due to the omnipresence of disorder or deviations from ideal models in real compounds. The spin-1/2 kagomé antiferromagnet (KAFM) is a canonical example of a frustrated system. An extensive search for a model compound has been carried out for the KAFM, so far mainly concentrating on copper minerals. In most of these, the valence state of Cu is 2+, giving the 3 d 9 electron configuration, meaning that the Cu 2+ ions carry spin-1/2. Furthermore, the Cu 2+ ion is usually coordinated by oxide or hydroxide ions in octahedral geometry. As a result of the strong Jahn-Teller effect in Cu 2+ , the degeneracy of Cu 3 d e g orbitals is always lifted, and either the d x2−y2 or d 3z2−r2 orbital is singly occupied: the d 3z2−r2 orbital is selected when two opposite Cu–O bonds are shorter than the other four bonds, whereas the d x2−y2 orbital is occupied when two Cu–O bonds are longer than the remainder. These orbitals overlap with nearby oxygen 2 p orbitals, giving rise to superexchange interactions between adjacent Cu 2+ spins. The balance between these interactions is particularly crucial for frustrated magnets, where small perturbations play a large role in determining the ground state. To give one example, in herbertsmithite ZnCu 3 (OH) 6 Cl 2 , the d x2−y2 orbital is selected by the Jahn-Teller distortion on each Cu 2+ ion, and arranged such that the crystallographic threefold axis is kept, resulting in spatially isotropic magnetic interactions within the kagomé layers [2] . No sign of long-range order has been observed in herbertsmithite down to 50 mK, despite a strong antiferromagnetic interaction of J= 170 K (refs 3 , 4 ). In the case of another Cu mineral, vesignieite, BaCu 3 V 2 O 8 (OH) 2 , the d 3z2−r2 orbital is selected and points towards the hydroxide ion located above the centre of a Cu triangle, resulting in an almost isotropic kagomé lattice with J avg =55 K (refs 5 , 6 , 7 ). We have thus far focused on volborthite Cu 3 V 2 O 7 (OH) 2 ·2H 2 O as a candidate for the spin-1/2 KAFM. In 1990, Lafontaine et al . [8] determined the crystal structure of volborthite by means of X-ray and neutron diffraction using polycrystalline samples. 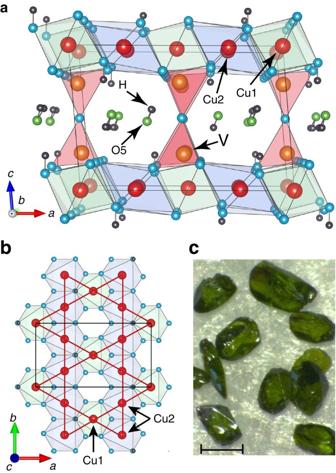Figure 1: Crystal structure of volborthite Cu3V2O7(OH)2·2H2O. (a,b) Crystal structure ofC2/mphase viewed along theb-axis (a) and perpendicular to theabplane. (b) The black line shows the unit cell, and the red lines highlight the kagomé lattice made up of Cu atoms. (c) Photograph of single crystals. Scale bar, 0.2 mm in length. Figure 1a,b depict Lafontaine's model, in which volborthite crystallizes in a monoclinic structure with the space group C 2/ m (No.12). The kagomé layer consists of edge-sharing CuO 6 octahedra and is separated by non-magnetic V 2 O 7 pillars and water of crystallization. There are two crystallographic sites for Cu; the Cu1 and Cu2 atoms form isosceles triangles with approximately 3% elongation, which are connected to each other to form a slightly distorted kagomé plane. Figure 1: Crystal structure of volborthite Cu 3 V 2 O 7 (OH) 2 ·2H 2 O. ( a , b ) Crystal structure of C 2/ m phase viewed along the b -axis ( a ) and perpendicular to the ab plane. ( b ) The black line shows the unit cell, and the red lines highlight the kagomé lattice made up of Cu atoms. ( c ) Photograph of single crystals. Scale bar, 0.2 mm in length. Full size image In volborthite, it is obvious from the deformations of the CuO 6 octahedra that the unpaired electrons on Cu1 and Cu2 occupy the d 3z2−r2 and d x2−y2 orbitals, respectively. As a result, there are two kinds of magnetic interactions: J 1 for Cu1-Cu2, and J 2 for Cu2-Cu2. The average of (2 J 1 + J 2 )/3 was estimated to be 77 K by a high-temperature series expansion fit of the magnetic susceptibility [9] . The nature of the magnetic ground state of volborthite has not been understood in detail yet, but is suggested to be unusual, with strong fluctuations at low temperature (LT) and short-range spin correlations [10] , [11] , [12] , [13] , [14] , [15] . One of the reasons for this ambiguity has been the unavailability of single crystals until now. In this study, we report a successful synthesis of single crystals of volborthite ( Fig. 1c ) for the first time. Single-crystal X-ray diffraction, magnetic susceptibility and heat capacity measurements were carried out, through which we established a unique structural transition at T s =310 K, whereby the orbital state of Cu1 switches from d 3z2−r2 at high temperature (HT) to d x2−y2 at LT. As a result, a complete magnetic long-range order is observed in the single crystal, apparently differing from the ground state previously reported for polycrystalline samples. 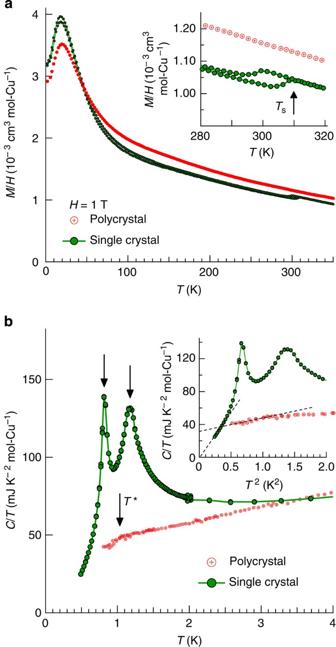Figure 2: Magnetic properties and heat capacity of single crystals of volborthite. (a) Temperature dependence of magnetic susceptibilities measured using an assembly of randomly oriented single crystals in a magnetic field of 1 T between 2 and 350 K upon cooling and heating. The data for a polycrystalline sample measured under the same conditions are plotted for comparison10. The data near room temperature (shown in the inset) reveals a first-order transition only for the single-crystal sample. (b) Temperature dependence of heat capacity divided by temperatureC/Tfor single and polycrystalline samples15measured below 4 K in zero magnetic field. Two peaks at 0.81 and 1.19 K are observed for the single-crystal sample instead of a kink atT*=1 K for the polycrystalline sample. The inset shows aC/TversusT2plot, in which the dotted lines are linear extrapolations towardsT=0. Magnetic properties Figure 2a shows the temperature dependence of the magnetic susceptibility measured upon both heating and cooling between 2 and 350 K under a magnetic field of 1 T. The measurements were performed for both a polycrystalline sample and a cluster of single crystals in arbitrary orientation. An anomaly is observed at ~300 K for the single crystals only, as shown in the inset of Fig. 2a ; their magnetic susceptibility suddenly increases by approximately 4×10 −5 cm 3 mol −1 Cu −1 at T s =310 K upon heating and decreases at 290 K upon cooling. The anomaly shows a distinct thermal hysteresis, indicating the occurrence of a first-order phase transition. The Weiss temperature, θ W , which measures the magnitude of net magnetic interactions, changes from −35 K at T > T s to −140 K at T < T s . This means that a large modification of the magnetic interactions in the kagomé plane takes place at the transition. Note, however, that both curves in Fig. 2a exhibit broad peaks at around ~20 K, suggesting similar development of short-range antiferromagnetic or singlet correlations at LTs. Figure 2: Magnetic properties and heat capacity of single crystals of volborthite. ( a ) Temperature dependence of magnetic susceptibilities measured using an assembly of randomly oriented single crystals in a magnetic field of 1 T between 2 and 350 K upon cooling and heating. The data for a polycrystalline sample measured under the same conditions are plotted for comparison [10] . The data near room temperature (shown in the inset) reveals a first-order transition only for the single-crystal sample. ( b ) Temperature dependence of heat capacity divided by temperature C / T for single and polycrystalline samples [15] measured below 4 K in zero magnetic field. Two peaks at 0.81 and 1.19 K are observed for the single-crystal sample instead of a kink at T * =1 K for the polycrystalline sample. The inset shows a C / T versus T 2 plot, in which the dotted lines are linear extrapolations towards T =0. Full size image Structural transition To investigate the transition at T s , X-ray diffraction experiments were carried out using a single crystal of dimensions 0.23×0.10×0.10 mm 3 . Superlattice reflections with half integer l for ( hkl ) reflections were observed below T s , indicating doubling of the unit cell along the c axis. The temperature dependences of the intensities of some superlattice reflections are shown in Fig. 3 . As they suddenly disappear at T s with increasing temperature, the anomaly observed at T s in magnetic susceptibility can be attributed to this structural phase transition. 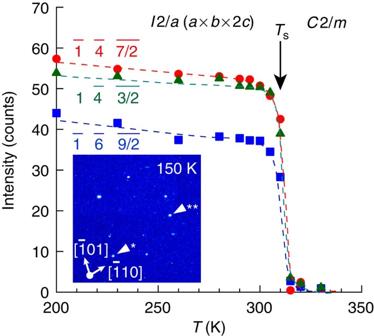Figure 3: First-order structural phase transition atTs. Temperature dependence of the intensity of superlattice reflections with indices −1 −4 −7/2, 1 −4 −3/2 and −1 6 −9/2 measured upon heating. The inset shows a CCD image obtained at 150 K, in which the arrows marked by * and ** show major superlattice reflections with indices of 7 8 1/2 and 5 10 1/2, respectively. Figure 3: First-order structural phase transition at T s . Temperature dependence of the intensity of superlattice reflections with indices −1 −4 −7/2, 1 −4 −3/2 and −1 6 −9/2 measured upon heating. The inset shows a CCD image obtained at 150 K, in which the arrows marked by * and ** show major superlattice reflections with indices of 7 8 1/2 and 5 10 1/2, respectively. Full size image Further single-crystal structural analyses were performed at 150 and 323 K to investigate the structural changes at T s . The HT phase has a monoclinic structure, with space group C 2/ m and lattice parameters of a =10.657(3) Å, b =5.887(1) Å, c =7.228(2) Å, and β =95.035(8)°. Structural refinements yielded essentially the same crystal structure as that reported by Lafontaine et al . [8] , with reliability factors R [ I >2σ( I )]=4.13% and w R 2=12.23%. The space group of the LT phase was determined to be I 2/ a (No. 15). The lattice parameters are a =10.6418(1) Å, b =5.8485(1) Å, c =14.4157(1) Å, and β =95.443(1)° at 150 K, and the resultant reliability factors R [ I >2σ( I )]=2.93% and w R 2=7.67%. The obtained structural data are provided in Supplementary Data 1 for the HT phase and Supplementary Data 2 for the LT phase. The position of hydrogen atoms could not be determined in the present analyses. Of primary interest is to understand how the structural phase transition modifies the Cu kagomé lattice and the environment around the Cu ions. The structures of the kagomé layer of both the HT and LT phases are depicted in Fig. 4a and b , respectively. As a result of the structural transition, a mirror plane and a twofold axis at the Cu1 site are lost with respect to the C 2/ m (HT) structure. This causes a large change in the coordination environment of the Cu1 site, including the O3 site splitting into two sites, O31 and O32. In the HT phase, the equatorial Cu1–O3 bonds (2.181(2) Å) are longer than the axial Cu1–O2 bonds (1.947(2) Å). When the transition occurs, two of the Cu1–O3 bonds are elongated by 7.2% to become Cu1–O31 bonds (2.3385(8) Å) and the other two are shortened by 9.0% to become Cu1–O32 bonds (1.9847(8) Å). These changes of the bond lengths are extraordinarily large, even discernible by eye in Fig. 4 . Note that there are four short bonds in the Cu1 octahedron in the LT phase, two Cu1–O2 and two Cu1–O32 and two long bonds, Cu1–O31. This means that the d x2−y2 orbital is selected in the LT phase, instead of the d 3z2−r2 orbital in the HT phase. On the other hand, the overall geometry of the Cu2 octahedron is preserved, with the Cu2–O31 bond elongating by 4.1% and the Cu2–O32 bond shrinking by 3.4%, such that the d x2−y2 orbital remains selected at LT. Thus, the spin-carrying orbital on both Cu 2+ sites is the d x2−y2 orbital in the LT phase, as in herbertsmithite. However, the orientations of the orbitals with respect to each other are different between the two compounds, and there is no threefold symmetry in the LT state of volborthite. 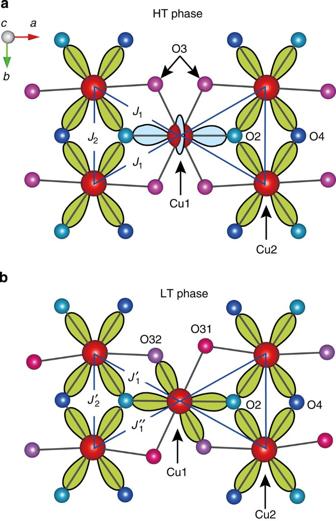Figure 4: Orbital switching transition of single crystal of volborthite. (a,b) Structure of the kagomé layer in the high-temperature (HT) phase (a) and the low-temperature (LT) phase (b). In the HT phase,d3z2−r2anddx2−y2orbitals are occupied by unpaired electrons at the Cu1 and Cu2 sites, respectively. In contrast,dx2−y2orbitals are selected at all the Cu sites in the LT phase, indicating that orbital switching takes place at the Cu1 site. Nearest-neighbour magnetic interactions change fromJ1andJ2in the HT phase toJ′1,J″1andJ′2in the LT phase. Figure 4: Orbital switching transition of single crystal of volborthite. ( a , b ) Structure of the kagomé layer in the high-temperature (HT) phase ( a ) and the low-temperature (LT) phase ( b ). In the HT phase, d 3z2−r2 and d x2−y2 orbitals are occupied by unpaired electrons at the Cu1 and Cu2 sites, respectively. In contrast, d x2−y2 orbitals are selected at all the Cu sites in the LT phase, indicating that orbital switching takes place at the Cu1 site. Nearest-neighbour magnetic interactions change from J 1 and J 2 in the HT phase to J ′ 1 , J ″ 1 and J ′ 2 in the LT phase. Full size image Phase transitions at LTs To investigate the physical properties of the single crystalline sample at LT, heat capacity measurements were carried out using an assembly of several single crystals ( Fig. 2b ). The C/T of the single crystals exhibits a sharp peak at 0.81 K and a relatively broad peak at 1.18 K, instead of the kink at 1 K observed previously for a polycrystalline sample [15] . These peaks are interpreted as two successive phase transitions, both probably of magnetic origin. Moreover, the T -linear term that is present in the polycrystalline sample is missing in the single-crystal sample, as shown in the inset of Fig. 2b . The change of orbital state found in volborthite should be distinguished from the phenomenon known as orbital ordering: in general, orbital order occurs in systems where the symmetry of the coordination polyhedra at elevated temperature is high, leading to orbital degeneracy. This symmetry may be broken, and a unique orbital configuration selected by a cooperative Jahn-Teller distortion at lower temperatures. For example, in NaNiO 2 (Ni 3+ , d 7 low spin), the unpaired electron occupies twofold degenerate e g orbitals at HT and selects the d 3z2−r2 orbital through an axial elongation of the NiO 6 octahedron below 480 K (ref. 16 ). Such a transition is an order–disorder transition associated with the orbital degree of freedom. Similar orbital ordering phenomena are observed in various 3 d transition metal compounds such as the perovskite manganite LaMnO 3 (ref. 17 ) and the vanadates ZnV 2 O 4 (ref. 18 ) or LiVO 2 ( [19] ). In contrast, because of the strong Jahn-Teller effect for the Cu 2+ ion, no corresponding orbital disordered state has been observed in copper compounds even at HT; most compounds decompose before orbital disordering. The change in the orbital state in volborthite, which occurs between two orbital ordered states, is thus not orbital order, but can instead be called orbital switching. To the best of our knowledge, this orbital switching has been observed for the first time. The origin of the orbital switching may be attributed to a change in hydrogen bonding between water molecules sandwiched by the kagomé layers and O3 (O31 and O32); the distances between O5 of the crystalline water and the O3 atoms are thus a means to estimate the strength of the hydrogen bonds. The O5–O3 distance in the HT phase (3.016(3) Å) is found to change into O5–O31 (2.944(2) Å) and O5–O32 (3.040(2) Å) in the LT phase. This shift is likely accompanied by orientational ordering of the crystalline water. To accommodate the stronger O5–H–O31 bond, O31 moves away from Cu1, resulting in O32 moving closer, and thus giving rise to the observed deformation of the CuO 6 octahedron. The reason why the orbital switching has been observed only for single crystals is unclear. One possibility is the presence of a nonstoichiometry of the crystalline water, which is more severe in polycrystalline samples. The apparent differences in the low-temperature physical properties between polycrystalline and single-crystal samples may be related to the presence of the orbital switching transition, as substantial changes in the magnetic interactions within the kagomé layers should result from the distortion of the Cu1 octahedron. In the HT phase, the d 3z2−r2 and d x2−y2 orbitals are occupied by unpaired electrons at the Cu1 and Cu2 sites, respectively, whereas d x2−y2 orbitals are selected at all the Cu sites in the LT phase. Therefore, the nearest-neighbour magnetic interactions should change from J 1 and J 2 in the HT phase to J ′ 1 , J ″ 1 and J ′ 2 in the LT phase, as shown in Fig. 4 . This reduction in symmetry may crucially affect the fragile magnetic ground states of the kagomé compounds, which are selected by a delicate balance of magnetic interactions within the kagomé plane. On the other hand, it is not clear whether the orbital switching transition is completely suppressed in a polycrystalline sample from its high-temperature properties. The change in magnetic interactions at T s gives rise to not only the reduction in symmetry of interactions but also the enhancement of antiferromagnetic correlation, which is evidenced by the change of Weiss temperature from θ W =−35 K in the HT phase to θ W =−140 K in the LT phase upon cooling. The Weiss temperature of the polycrystalline sample is θ W =−105 K, which is in between those of the LT and HT phases in a single crystal, albeit closer to the former. This suggests that the orbital switching transition takes place at least partially in a polycrystalline sample, although it is not discernible as a transition in the magnetic susceptibility data of Fig. 2a . As mentioned previously, the undistorted compound herbertsmithite shows no transition to a magnetic frozen state down to 50 mK at low magnetic fields [4] , consistent with predictions for the spin-1/2 KAFM. It does, however, exhibit a field-induced freezing above a critical field of 1.6 T (ref. 20 ). In contrast, the off-stoichiometric so-called paratacamites of formula Zn x Cu 4− x (OH) 6 Cl 2 assume partly frozen states at LT, with two magnetic transitions finally observed at 18.1 and 6.5 K for the end member ( x =0), clinoatacamite [4] , [21] , [22] , [23] . The tendency to magnetic order in paratacamites may be induced by interplane couplings through Cu defect spins at the Zn site between the kagomé layers, as well as the likely presence of a sizable Dzyaloshinsky-Moriya term. On the other hand, the nearly undistorted kagomé compound vesignieite, BaCu 3 V 2 O 8 (OH) 2 , has recently been reported to show a peculiar transition at 9 K to a partly frozen state with persisting spin dynamics [6] , [7] , despite no order being found in previous studies [5] . It is suggested that this order occurs owing to a large Dzyaloshinsky-Moriya interaction within the kagomé plane [6] , [7] . The examples of paratacamites and vesignieite expose the diversity of the physics which emerge when the KAFM is perturbed. Our work on volborthite increases the range of possibilities further, with several unique features observed in our experiments: the presence of two phase transitions; the large ratio of Weiss constant to the transition temperature (>100 versus ~6 for vesignieite); and the enhancement of the transitions as crystallinity is improved. The challenge now remains to clarify the delicate interplay of perturbations that determine the mysterious ground state of volborthite, and particularly the role of the orbital switching transition. This will be a joint effort between experiment using techniques such as NMR, μSR (muon spin rotation, relaxation, resonance) and neutron scattering, as well as theory. It is hoped that the investigation will also shed light on the peculiar ordered states observed in other kagomé compounds, and maybe even give an insight into the physics of the pure KAFM. In summary, high quality single crystals of the spin-1/2 quasi-KAFM volborthite, Cu 3 V 2 O 7 (OH) 2 ·2H 2 O, were successfully synthesized. We found a first-order structural phase transition at T s =310 K, which has not yet been observed in polycrystalline samples. This structural transition is caused by orbital switching at the Cu1 site from the d 3z2−r2 to the d x2−y2 orbital at T s upon cooling. Magnetic long-range order occurs through two successive phase transitions at around 1 K in single crystals, which apparently differs from the LT behaviour of polycrystalline samples. Sample preparation In previous studies, polycrystalline samples were obtained by a precipitation, and subsequent heat treatment under hydrothermal conditions [10] . The maximum particle size obtained by this method was on the order of a few micrometers. We prepared single crystals of volborthite of submilimeter size by a direct reaction of Cu(OH) 2 and V 2 O 5 under hydrothermal conditions: 2.342 g of Cu(OH) 2 (99% purity) and 1.455 g of V 2 O 5 (99.99%) in a molar ratio of 3:1 with 15 ml of 1% HNO 3 aqueous solution were put in a Teflon beaker of φ 2.8×3.5 cm 3 size and 27 ml in volume, which was placed in a steel autoclave. The autoclave was heated to 180 °C at a rate of 1 °C min −1 , kept there for 3 h and cooled to 130 °C at a rate of 0.33 °C h −1 . Green single crystals of maximum size 0.7 mm, such as those shown in Fig. 1c , were obtained. Structural analysis X-ray diffraction experiments were carried out using a single crystal of dimensions 0.23×0.10×0.10 mm 3 . They were carried out on a triple-axis diffractometer (SMART APEX with a CCD detector, Bruker) using Mo-K α radiation. Diffraction intensities were measured at temperatures between 150 and 330 K using the SAINT program and corrected for absorption using the SADABS software [24] . The charge flipping method was applied to decide initial structural parameters [25] . Structural parameters were refined using the program SHELXL based on the full-matrix method [26] . Anisotropic displacement parameters were assumed for all non-hydrogen atoms. Several single crystals were examined and found to show the same orbital switching transition from the C 2/ m to I 2/ a structure below T s . Magnetic susceptibility and heat capacity measurements Magnetic susceptibility data were collected using a SQUID magnetometer (Quantum Design MPMS). Heat capacity measurements were carried out by the heat-relaxation method in a Quantum Design PPMS. We measured heat capacity on several batches of single crystals to secure the reproducibility and observed essentially the same two-step transitions at nearly equal temperatures, although the sharpness of the peaks changed slightly from sample to sample. How to cite this article: Yoshida, H. et al . Orbital switching in a frustrated magnet. Nat. Commun. 3:860 doi: 10.1038/ncomms1875 (2012).